Sea-level variability over five glacial cycles Research on global ice-volume changes during Pleistocene glacial cycles is hindered by a lack of detailed sea-level records for time intervals older than the last interglacial. Here we present the first robustly dated, continuous and highly resolved records of Red Sea sea level and rates of sea-level change over the last 500,000 years, based on tight synchronization to an Asian monsoon record. We observe maximum ‘natural’ (pre-anthropogenic forcing) sea-level rise rates below 2 m per century following periods with up to twice present-day ice volumes, and substantially higher rise rates for greater ice volumes. We also find that maximum sea-level rise rates were attained within 2 kyr of the onset of deglaciations, for 85% of such events. Finally, multivariate regressions of orbital parameters, sea-level and monsoon records suggest that major meltwater pulses account for millennial-scale variability and insolation-lagged responses in Asian monsoon records. Sea-level change is a primary diagnostic indicator of global ice-volume variability, a key feedback process in climate change. Radiometrically dated relative sea-level (RSL) indicators—such as fossil corals, submerged speleothems and palaeoshoreline deposits—provide strong constraints on sea-level (ice-volume) reconstructions. However, before ~150,000 years (~150 kyr) ago, such data are scarce and are largely limited to interglacials, which renders them unsuitable for portraying the timing, amplitude and rates of older sea-level changes. Alternatively, ice-volume changes can be approximated using benthic foraminiferal δ 18 O, but this approach is compromised by poorly understood deep-water temperature influences [1] , and variable spatial gradients in benthic δ 18 O (refs 2 , 3 ). Here we address the above issues with a new chronology derived from a U/Th-dated speleothem δ 18 O record, for a continuous, high-resolution record of Red Sea RSL [4] over five complete glacial cycles (500 kyr). Our new approach relies on synchronizing a distal monsoon signal with both dust and sea-level records; hence, it employs different criteria than the recent age model development for this record over the youngest 150 kyr (ref. 5 ). That approach, which correlated (proximal) source-water and sea-level-equivalent δ 18 O records, achieved smaller uncertainties, but could not be extended to older ages ( Supplementary Note 1 ). We link our new chronology over the older interval (150–500 kyr) to previous results for the last 150 kyr (ref. 5 ). By transferring a U/Th chronology to the entire 500 kyr Red Sea RSL record, and propagating quantifiable sources of uncertainty, we can investigate how the global glaciation state (total ice volume) affects potential maximum rates of sea-level rise. An additional (major) benefit is that it provides the first chronologically independent sea-level record for future investigations of ice-volume phasing relative to insolation (orbital) and polar climate forcing over multiple glacial cycles. Finally, we synchronize an Asian dust-flux signal with our new chronology; hence, our final dataset comprises records of sea-level change and Asian summer and winter monsoon intensity on the same timescale, spanning five complete glacial cycles. Although many hypotheses exist regarding connections between changes in ice volume and monsoon intensity [6] , [7] , [8] , detailed understanding of this relationship is lacking [9] , [10] . This is partly due to the fact that previous hypotheses relied on benthic δ 18 O ice-volume proxies and/or poorly defined ice sheets in monsoon models [9] , [11] . Our approach improves the capacity to distinguish the relative impacts of orbital forcing, ice volume and rates of ice-volume change on monsoon variability. Age model development Our chronology is developed in two stages. First, we synchronize Red Sea dust-flux data ( Fig. 1b ) with positive (U/Th-dated) δ 18 O anomalies, or weak monsoon events, within glacial terminations in Sanbao Cave, China (δ 18 O sanbao ) [8] , [12] ( Fig. 1a , Supplementary Fig. 1 ). Dust-flux data for central Red Sea core KL09 comprise Ti/Ca ratios and hematite (‘Hem’) abundance from the same sediment samples as the RSL data so that timing relationships are unambiguous [13] , [14] ( Supplementary Note 1 , Supplementary Fig. 2 ). All five glacial terminations (T1–T5) contain a large mid-termination dust peak, followed by a sharp drop toward the subsequent interglacials ( Fig. 1b,c ). Striking signal similarity between Red Sea and Asian dust records suggests covariation in dust mobilization over these regions due to large-scale atmospheric circulation changes [14] . This is corroborated by dependence of Red Sea dust fluxes on seasonal wind changes associated with Indian monsoon circulation [15] , which is closely coupled with East Asian monsoon dynamics [16] , [17] . We therefore hypothesize that a close relationship exists between weak monsoon events in Sanbao Cave and Red Sea dust spikes during glacial terminations. We test this hypothesis by correlating KL09 Ti/Ca to δ 18 O sanbao at T1 to T5 ( Fig. 1a,b ), transferring this age model (with linear interpolation between terminations) to the RSL data (‘RSL dust-Sanbao ’, Fig. 1c ), and then comparing the inferred timing of major sea-level rises in RSL dust-sanbao with that determined from 40 Ar/ 39 Ar-dated ash (tephra) layers deposited within sea-level-controlled sedimentary sequences from coastal plains of the Palaeo-Tiber River, Italy [18] , [19] ( Supplementary Note 2 , Supplementary Figs 3–5 , Supplementary Table 3 ). The inferred timing of T3 and T5 from our dust-δ 18 O sanbao correlation closely matches that of aggradational units from the Palaeo-Tiber River ( Fig. 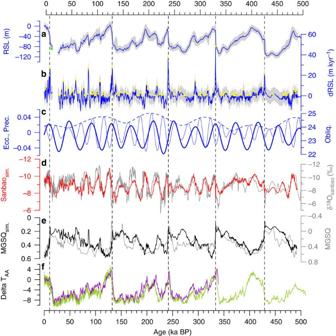Figure 3: Sea-level and orbital time series with simulated Asian monsoon records. (a) Red Sea RSL record (fromFig. 2) (probability maximum, blue; 95% confidence interval of the RSL dataset, light grey). (b) Rates of RSL change (dRSL, blue; ±2σ, grey) with marked points ofFig. 4dRSL data (yellow dots) and MWP-1a (green dot). (c) Eccentricity (E, dashed), precession (P, hairline) and obliquity (O, solid)56. (d) δ18Osanbao(grey) and MLR simulation of δ18Osanbao(red). (e) Grain-size record from the Chinese Loess Plateau (MGSQ, grey34) and MLR simulation of MGSQ (black). (f) Antarctic temperature (green20, purple26). Vertical dashed lines indicate peak sea-level rise rates at glacial terminations. 1c ). Further validation of our hypothesis is provided by good agreement between RSL dust-Sanbao and the same RSL data on an independently constrained chronology for 0–150 kyr (ref. 5 ) (‘RSL 150 ’, Fig. 1c ). 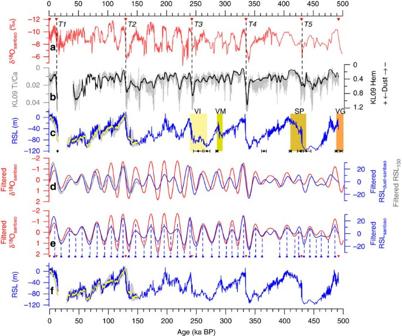Hence, we retain the ‘dust-Sanbao’ synchronization. Figure 1: Synchronization of Red Sea dust and RSL records with Asian speleothem δ18O. (a) Sanbao Cave speleothem δ18O. (b) Red Sea core KL09 dust proxies (Ti/Ca, grey; hematite concentration (Hem), black). Correlation ties (dashed lines, red triangles) at glacial terminations (T1–T5) are indicated. (c) Red Sea RSL record after the dust-Sanbao synchronization (blue), and on an independent chronology (95% confidence intervals, grey; probability maximum, yellow).40Ar/39Ar tephra datings (black dots with 2σerror bars) within Palaeo-Tiber River aggradational units VI (Vitinia Formation), VM (Via Mascagni parasequence), SP (San Paolo Formation), and VG (Valle Giulia Formation)18,19(coloured rectangles) are indicated (seeSupplementary Note 2andSupplementary Figs 3–5). (d,e) 22 kyr band-pass-filtered records of δ18Osanbao(red), RSLdust-sanbao(blue) and RSL150(yellow) before (d) and after (e) synchronization at 17 tie-points (blue triangles ine). (f) Red Sea RSL record (blue) after synchronizations shown inb,e, and on an independent chronology (as inc). RSL and KL09 records are not reliableca.14–23 ka and 14–40 ka, respectively, due to an indurated aplanktonic interval. Figure 1: Synchronization of Red Sea dust and RSL records with Asian speleothem δ 18 O. ( a ) Sanbao Cave speleothem δ 18 O. ( b ) Red Sea core KL09 dust proxies (Ti/Ca, grey; hematite concentration (Hem), black). Correlation ties (dashed lines, red triangles) at glacial terminations (T1–T5) are indicated. ( c ) Red Sea RSL record after the dust-Sanbao synchronization (blue), and on an independent chronology (95% confidence intervals, grey; probability maximum, yellow). 40 Ar/ 39 Ar tephra datings (black dots with 2 σ error bars) within Palaeo-Tiber River aggradational units VI (Vitinia Formation), VM (Via Mascagni parasequence), SP (San Paolo Formation), and VG (Valle Giulia Formation) [18] , [19] (coloured rectangles) are indicated (see Supplementary Note 2 and Supplementary Figs 3–5 ). ( d , e ) 22 kyr band-pass-filtered records of δ 18 O sanbao (red), RSL dust-sanbao (blue) and RSL 150 (yellow) before ( d ) and after ( e ) synchronization at 17 tie-points (blue triangles in e ). ( f ) Red Sea RSL record (blue) after synchronizations shown in b , e , and on an independent chronology (as in c ). RSL and KL09 records are not reliable ca. 14–23 ka and 14–40 ka, respectively, due to an indurated aplanktonic interval. Full size image Next, we ‘fine-tune’ the dust-tuned RSL record by adding age control between the dust:Sanbao ties. Cross-spectral phase analyses of Ti/Ca dust-sanbao and RSL dust-sanbao with δ 18 O sanbao reveal strong covariance in the precession band ( Supplementary Fig. 6b,c ), particularly between RSL dust-sanbao and δ 18 O sanbao (90% coherent; Supplementary Note 1 ). Application of a 22-kyr band-pass filter to all three records reveals that precession-band variance is broadly in phase (within 2–3 kyr) between RSL and δ 18 O sanbao , which is corroborated when using the independently dated RSL 150 (ref. 5 ) instead of RSL dust-sanbao ( Supplementary Fig. 6d ). Visual comparison of precession-band variance in RSL 150 and δ 18 O sanbao confirms that offsets are minor (within ±1 kyr) and not systematic in direction or magnitude ( Fig. 1d ). In contrast, phasing of comparable peaks in the filtered Ti/Ca and δ 18 O sanbao records varies by −180 to +180° within a single glacial cycle, and has no systematic trend among successive glacial cycles ( Supplementary Fig. 7 ). We therefore exploit the highly consistent precession-band covariance between RSL dust-sanbao and δ 18 O sanbao to improve our RSL dust-sanbao chronology for 150–500 kyr. At maximum coherency (equivalent to a frequency of 0.045 kyr −1 ), phase offsets between δ 18 O sanbao and RSL dust-sanbao are −2.7±0.4 kyr, but just −0.4±1 kyr when we use RSL 150 ( Supplementary Fig. 6b,d ). Age control in RSL 150 is superior to that in RSL dust-sanbao , so the precession-band δ 18 O sanbao -RSL phasing inferred from RSL 150 should be far more accurate than that inferred from RSL dust-sanbao . On the basis of this, we apply a 0.045 kyr −1 band-pass filter to δ 18 O sanbao and RSL dust-sanbao ( Supplementary Fig. 7 ), and then synchronize peaks and troughs in the filtered δ 18 O sanbao and RSL dust-sanbao records ( Fig. 1e ). We assume that the precession-band δ 18 O sanbao -RSL phasing inferred from RSL 150 applies to intervals between terminations of previous glacial cycles ( Fig. 1d,e ). Within uncertainties, this is likely a reasonable assumption, given that the relationship between key climate-system variables (methane, temperature and CO 2 ) is consistent over (at least) eight glacial cycles [20] . We also emphasize that, because ice-volume phase relationships at terminations were likely dependent on ice volume at the preceding glacial maximum, we maintain the dust-Sanbao synchronization to date terminations ( Fig. 1a,b ), and synchronize RSL dust-sanabo and δ 18 O sanbao solely between terminations ( Fig. 1d,e ). Linear interpolation between these (‘fine-tune’) tie-points yields ‘RSL sanbao ’, with age control every ~11 kyr ( Fig. 1f ). Our fine-tuning approach is validated by improved agreement of RSL 150 and RSL sanbao , compared with RSL 150 and RSL dust-sanbao ( Fig. 1c,f ). Uncertainty propagation We now account for all uncertainties that can be reasonably quantified, associated with the dust-Sanbao and RSL-Sanbao correlations between 150 and 500 kyr. (We use RSL 150 for the 0–150 kyr interval, for which a thorough uncertainty propagation and probabilistic assessment has already been established [5] ). Sources of uncertainty are: U/Th-dating, sample-spacing in the δ 18 O sanbao and KL09 Ti/Ca records, peak detection in the filtered δ 18 O sanbao and RSL dust-sanbao records, and phasing between precession-band covariance in δ 18 O sanbao and RSL dust-sanbao . While there might be a systematic phase drift between Southeast Asian water isotopes and Red Sea RSL over time, this cannot be adequately constrained at present so we do not attempt to include it in our error propagation. To determine U/Th-dating uncertainties for every tie-point, we use ‘OxCal’ software (version 4.2 (refs 21 , 22 )) to apply a Bayesian deposition model to each of the eight stalagmites used in the original Sanbao Cave chronology ( Supplementary Table 1 ). The advantage of a Bayesian approach is that it accounts for increased chronological uncertainty between dated horizons in a depositional sequence, hence it is far more robust than employing straightforward linear interpolations. Further technicalities of OxCal and application of Bayesian tools in age modelling are detailed elsewhere [21] , [22] , [23] , [24] . There is no significant difference between the original Sanbao chronology [8] , [12] , [25] and our Bayesian model output ( Supplementary Fig. 8 ) so, given the wide usage of the Sanbao chronology, it is more convenient in relation to other published material to maintain the original δ 18 O sanbao chronology on which our correlations are based, and use Bayesian modelling solely for uncertainty estimation ( Supplementary Note 1 ). The accuracy of our new RSL chronology also depends on how confidently we can detect peaks/troughs in the precession-band-filtered δ 18 O sanbao and RSL dust-sanbao records. We therefore follow an approach similar to Kawamura et al . [26] by adding white noise to the δ 18 O sanbao and RSL dust-sanbao records (based on 2 s.d. errors of ±12 m for Red Sea RSL [4] , [27] and ±0.16‰ for δ 18 O sanbao (ref. 25 )) to generate 1,000 artificial datasets; we then identified peaks in the precession-band-filtered artificial data to determine the mean and variance associated with the age of each peak in the original record. Every simulation captures all precession-band peaks/troughs over the past 500 kyr ( Supplementary Fig. 7 ), and the simulated data scatter gives a reliable estimate of peak-detection uncertainties ( Supplementary Table 1 ). We established above that precession-band phase offsets between δ 18 O sanbao and RSL 150 are −0.4±1.0 kyr (at 2 σ ); we therefore use a 1-kyr phase-offset uncertainty in our error propagation. All uncertainties are finally combined in a root mean square calculation ( Supplementary Table 1 ). These fully propagated tie-point uncertainties are then coupled with the RSL sanbao time series in a Bayesian deposition model (again using OxCal) to statistically interpolate a chronological uncertainty for every RSL sanbao datapoint ( Supplementary Fig. 9 ). Red Sea RSL variability To complete our RSL reconstruction, we combine synchronization (age) uncertainties between 150 and 500 kyr with sea-level uncertainties (±12 m at 2 σ (refs 4 , 27 )) in a Monte Carlo-style probabilistic assessment (Methods). Coupling these new results to previous results for RSL 150 (ref. 5 ) gives a complete probabilistic assessment of Red Sea RSL over the last 500 kyr ( Fig. 2 ; Supplementary Data 1 ). Chronological agreement between RSL and U/Th-dated coral and speleothem sea-level information for the intervals 0–150 kyr (ref. 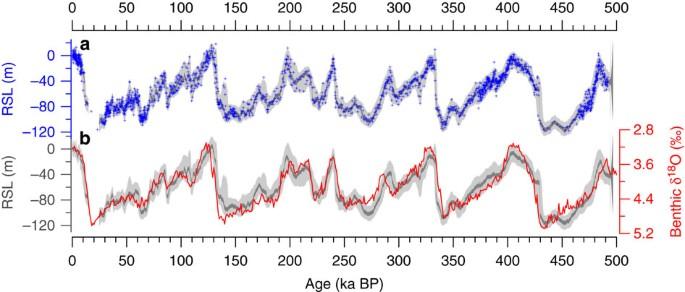5 ) and 150–500 kyr ( Supplementary Fig. Figure 2: Radiometrically constrained 500 kyr RSL record with fully propagated uncertainties. (a) Red Sea RSL data (blue) for 0–150 kyr (ref.5) and 150–500 kyr (this study), superimposed on the 95% probability interval of the RSL dataset (light grey) and 95% probability interval for the probability maximum (dark grey). (b) Probabilistic RSL record as ina, but with superimposed (red) benthic foraminiferal δ18O (ref.28). 10 ), corroborates the timing of sea-level highstands inferred from our RSL record ( Supplementary Table 2 ). RSL and global benthic δ 18 O variations [28] are also broadly similar ( Fig. 2 ), but phase and amplitude offsets exist that require removal of the temperature component from benthic δ 18 O (ref. 1 ). Figure 2: Radiometrically constrained 500 kyr RSL record with fully propagated uncertainties. ( a ) Red Sea RSL data (blue) for 0–150 kyr (ref. 5 ) and 150–500 kyr (this study), superimposed on the 95% probability interval of the RSL dataset (light grey) and 95% probability interval for the probability maximum (dark grey). ( b ) Probabilistic RSL record as in a , but with superimposed (red) benthic foraminiferal δ 18 O (ref. 28 ). Full size image It is pertinent to briefly discuss the extent to which the Red Sea RSL record approximates global (eustatic) sea level (ESL). RSL reconstructions are, by definition, representative of sea-level changes at a particular geographic location. Any isostatic and tectonic effects on site elevation will result in deviations of the respective ‘uncorrected’ RSL signal from ESL. The Red Sea RSL record technically represents sea-level fluctuations at Hanish Sill (RSL HS ), the hydraulically limiting ridge at the southern entrance to the Red Sea. Isostatic changes in Hanish Sill depth are implicitly accounted for in the hydraulic model used to convert Red Sea δ 18 O to sea level, by scaling the model to the ESL glacial–interglacial range indicated by coral sea-level data [29] . Tectonic changes have been considered in the Red Sea RSL model [29] and are supported by subsequent work [30] , which concluded that vertical tectonic stability characterized the Hanish Sill region for at least the past 120 kyr. Modelling the isostatic response of Hanish Sill using a global ice model (ICE-5G) [31] implies that, while the relationship between RSL at Hanish Sill (RSL HS ) and ESL varies in detail over time, RSL HS generally scales proportionally with land-ice variations ( Supplementary Fig. 11 ). The offset between RSL HS and ESL is greatest at glacial maxima (~8–20%, considering all Earth model outputs). For example, regarding the last glacial maximum (=26 kyr in the model output), the modelled RSL HS and ESL ranges are −105.6 to −123.3 m and −132.4 to −134.3 m, respectively ( Supplementary Fig. 11 ). The RSL HS :ESL relationship also appears to depend on the phase of the glaciation–deglaciation cycle ( Supplementary Fig. 12 ): larger RSL HS :ESL offsets are observed for deglaciations compared to glaciations. To explore the potential effect of these pathways on the relationship between RSL HS and ESL change rates (dRSL HS , dESL), we compared modelled dRSL HS and dESL for a range of Earth models (including variable lithospheric thicknesses and mantle viscosities). Modelled dRSL HS and dESL vary in concert and are strongly correlated ( Supplementary Fig. 13 ). While the choice of Earth model slightly modifies absolute values, there is no apparent time lag between modelled dRSL HS and dESL ( Supplementary Fig. 13a ). This suggests that observed hysteresis in RSL HS :ESL glaciation/deglaciation pathways does not affect RSL HS and ESL change rates, and instead simply relates to the (variable) scaling factor between RSL HS and ESL. Maximum rates of sea-level rise Following a similar probabilistic approach as Grant et al . [5] , we determine rates of sea-level change (dRSL) over the last 500 kyr ( Fig. 3b ; Supplementary Data 1 ). Our method involves a 500-year Gaussian smoothing of each RSL realization, so resultant dRSL values may conceal shorter periods of higher rates of sea-level change. Smoothing the RSL record before calculating its derivative with respect to time is necessary because sample-to-sample noise, inherent in any time series, would otherwise be amplified in the resultant dRSL record; hence, that record would be biased toward higher amplitudes. Equally, smoothing will underestimate dRSL when RSL changes abruptly. The sampling interval in the RSL record is approximately one sample per ~200 years, so our 500-year smoothing optimizes the balance between competing smoothing biases: a narrower smoothing window would place too much emphasis on individual datapoints, and a wider window would not accurately capture higher amplitude change rates. Figure 3: Sea-level and orbital time series with simulated Asian monsoon records. ( a ) Red Sea RSL record (from Fig. 2 ) (probability maximum, blue; 95% confidence interval of the RSL dataset, light grey). ( b ) Rates of RSL change (dRSL, blue; ±2 σ , grey) with marked points of Fig. 4 dRSL data (yellow dots) and MWP-1a (green dot). ( c ) Eccentricity (E, dashed), precession (P, hairline) and obliquity (O, solid) [56] . ( d ) δ 18 O sanbao (grey) and MLR simulation of δ 18 O sanbao (red). ( e ) Grain-size record from the Chinese Loess Plateau (MGSQ, grey [34] ) and MLR simulation of MGSQ (black). ( f ) Antarctic temperature (green [20] , purple [26] ). Vertical dashed lines indicate peak sea-level rise rates at glacial terminations. Full size image Extension of the dRSL record from one to five glacial cycles allows well-constrained assessment of the relationship between maximum ‘natural’ (preanthropogenic forcing) rates of sea-level rise and ‘glaciation state’, where the latter is defined as past global ice volume (approximated here by RSL, after conversion into equivalent ESL values; Supplementary Fig. 12a ) relative to present-day global ice volume (equivalent to ~65 m ESL; Supplementary Data 2 ). We also define deglaciation ‘events’ and ‘pulses’, whereby a deglaciation event is an interval of continuous positive dRSL values, and a ‘deglaciation pulse’ is a spike of maximum dRSL (within a deglaciation event) that immediately succeeds a negative inflection in the dRSL record ( Supplementary Fig. 14 ). Uncertainties in sea-level rise rates are taken from Fig. 3b , and glaciation-state uncertainties are taken from Supplementary Fig. 12a . For every deglaciation event/pulse in the past 500 kyr, we compare relative ice volume at the start of each event/pulse with the maximum sea-level rise rates per event/pulse ( Fig. 3b , Fig. 4a,b ). We also include values for meltwater pulse (MWP) 1a (4.6±0.6 m per century (m cy −1 ), based on U/Th-dated corals from offshore Tahiti) [32] , which was a well-documented, rapid sea-level rise during the last deglaciation. Our data suggest that, for both ‘event’ and ‘pulse’ scenarios, natural rise rates do not exceed ~2 m cy −1 and are mostly ≤1 m cy −1 for ice volumes up to about twice as large as present-day values ( Fig. 4a,b ). For larger ice volumes, substantially higher rise rates may be attained. The highest value (4.0–5.7 m cy −1 at 95% confidence limits) corresponds to termination 4 (T4) at ~334 kyr ( Fig. 3b ). In comparison, MWP-1a is not exceptional, especially in view of the 0.5-kyr smoothing in our method. 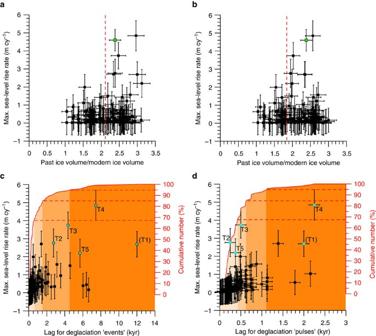Figure 4: Deglaciation episodes in the last 500 kyr. Maximum sea-level rise rates are plotted against: (a,b) relative ice volume at the start of a deglaciation event (a) and pulse (b) and (c,d) lag between the onset of deglaciation events (c) and pulses (d) and peak sea-level rise rates. Inferred ice-volume thresholds (red dashed lines) and MWP-1a (green32) are shown ina,b. The cumulative distribution of the number of deglaciation events/pulses as a function of lag is shown inc,d(solid red line), where the 68, 85 and 95% levels (red dashed lines) and corresponding lag intervals (orange shadings) are indicated. All error bars denote ±2σ. Horizontal error bars incare not visually detectable. Figure 4: Deglaciation episodes in the last 500 kyr. Maximum sea-level rise rates are plotted against: ( a , b ) relative ice volume at the start of a deglaciation event ( a ) and pulse ( b ) and ( c , d ) lag between the onset of deglaciation events ( c ) and pulses ( d ) and peak sea-level rise rates. Inferred ice-volume thresholds (red dashed lines) and MWP-1a (green [32] ) are shown in a , b . The cumulative distribution of the number of deglaciation events/pulses as a function of lag is shown in c , d (solid red line), where the 68, 85 and 95% levels (red dashed lines) and corresponding lag intervals (orange shadings) are indicated. All error bars denote ±2 σ . Horizontal error bars in c are not visually detectable. Full size image Further insight is gained by considering the lag between the onset of sea-level rise and the time of peak rise rates, for both deglaciation ‘events’ ( Fig. 4c ) and ‘pulses’ ( Fig. 4d ) ( Supplementary Table 4 ). In both cases, longer (shorter) lags tend to be associated with higher (lower) sea-level rise rates, but this is not always the case. Our data also show that while ‘ramping up’ periods–from the start of deglaciation to maximum melting–may last for several millennia (up to ~8 kyr, excluding the less reliable value for T1), they may also be considerably shorter (for example, ~3 kyr for T2; Fig. 4c ). Furthermore, a large proportion (85%) of all melting episodes reaches maximum sea-level rise rates within 1.5 kyr ( Fig. 4c ), and the final melting ‘pulse’ within a deglaciation episode is rapid relative to the ramping up period (≤0.6 and ≤1.1 kyr lag for 85 and 95% of cases, respectively; Fig. 4d ; Supplementary Table 4 ). Such observations provide important constraints for validating model-based assessments of ice-volume variability. Clearly, our observations of sea-level rise rates depend on the smoothing function applied to each RSL realization. However, as explained above, if smoothing is too low/high our conclusions will not be robust. Nevertheless, for completeness, we repeated our sea-level rise analyses for 250, 375, 750, 1,000 and 2,000-year smoothings ( Supplementary Figs 15–17 ). A straightforward comparison of sea-level rise rates at glacial terminations, based on different smoothings ( Supplementary Fig. 18 ), shows that the 2,000-year smoothing fails to capture real variations between termination rise rates ( Supplementary Fig. 15 ). Considering, therefore, the 250−1,000-year smoothings, we find that our ice-volume ‘threshold’ observation (that is, natural rise rates do not exceed ~2 m cy −1 and are mostly ≤1 m cy −1 for ice volumes up to twice as large as present-day values) holds irrespective of smoothing function ( Supplementary Fig. 16 ). The effect of different smoothings is far more apparent in our lag analyses. For example, for 85% of deglaciation events/pulses, the difference between a 250- and 1,000-year smoothing is an eight-/sixfold lag increase ( Supplementary Table 4 ). However, if we consider the less extreme 375- and 750-year smoothings, the lag difference is two- to threefold. Regardless, it is to be expected that lags quantified using time-derivative records will be strongly dependent on smoothing of the original time series. Given that the 250-/1,000-year smoothings yield considerably larger/smaller dRSL values than the 500-year smoothing, and that the 500-year smoothing is preferable for the sampling resolution of the original RSL time series, the 250-/1,000-year smoothings will likely under/overestimate lags in our analyses. Ice-volume and monsoon variability Ice-sheet changes and monsoon circulation are important for Earth’s radiative budget and internal energy redistribution. However, process understanding of interactions between these climate-system components remains elusive because of a lack of consistent age control among long records of ice-volume and monsoon variability. We have synchronized RSL with δ 18 O sanbao , a proxy for Asian summer monsoon (ASM) intensity [8] . Roberts et al . [14] demonstrated a close relationship between Red Sea dust and Chinese loess deposition, a proxy for Asian winter monsoon (AWM) intensity [33] , as measured by mean grain-size of quartz (MGSQ) [34] . Hence, we can transpose our new chronology to MGSQ ( Supplementary Note 3 , Supplementary Fig. 19 , Supplementary Table 5 , Supplementary Data 3 ) to investigate whether past ice-volume changes affected ASM and AWM intensity, as previously inferred for both orbital and suborbital timescales [6] , [17] , [35] . We assess the extent to which orbital forcing, ice-volume variations (RSL) and/or rates of ice-volume change (dRSL) may account for three key aspects: first, the amplitude of ASM fluctuations (δ 18 O sanbao ) (refs 8 , 12 ); second, the lag between insolation changes and δ 18 O sanbao ; and third, the timing and amplitude of AWM fluctuations (MGSQ) (ref. 34 ). We use multiple linear regressions (MLRs) to evaluate which combinations of orbital parameters (eccentricity, precession and obliquity; EPO), RSL and dRSL best agree with δ 18 O sanbao and MGSQ ( Fig. 3d,e ). Our MLR ‘simulation’ of δ 18 O sanbao (Sanbao sim ; Supplementary Data 3 ) explains 36% of the variance in δ 18 O sanbao compared with 21% explained by EPO alone, with both RSL and dRSL being significant components ( Fig. 3d ; Supplementary Fig. 20 , Supplementary Table 6 ). Sequential addition of the components in Sanbao sim reveals that ASM variations are paced predominantly by orbital forcing, slightly amplitude modulated by ice volume, and become lagged due to rapid ice-volume change ( Supplementary Fig. 21a –c) (see below). The combined orbital components within Sanbao sim have nearly identical variance to boreal mid-summer insolation ( Supplementary Fig. 21a ), as may be expected if δ 18 O sanbao reflects (at least in part) summer insolation-forced ASM variability [8] . However, the simulated orbital component is not directly in phase with δ 18 O sanbao , and cross-spectral phase analyses of δ 18 O sanbao with the permutations of Sanbao sim (for example, orbital components alone, orbital components plus RSL and so on) reveal that the phase offsets seen between δ 18 O sanbao and insolation (EPO) alone are reduced by ~20–40% when ice-volume effects (RSL and dRSL components) are included ( Supplementary Table 7 ). Our MLR simulation of the Chinese loess MGSQ record (MGSQ sim ; Supplementary Data 3 ) shares 44% of variance with MGSQ and is dominated by RSL (37% of variance), with minimal contribution from orbital components ( Fig. 3e ; Supplementary Figs 20 and 21 , Supplementary Table 6 ). A weak dRSL component in MGSQ sim principally accentuates dust-flux maxima at glacial terminations ( Fig. 3e , Supplementary Fig. 21f ). The slight yet significant contribution of the dRSL component to both Sanbao sim and MGSQ sim is confirmed by sensitivity tests ( Supplementary Fig. 20 ; Methods Section), which show that inclusion of dRSL not only improves the fit of the δ 18 O sanbao and MGSQ MLR models, it also–more importantly–improves model prediction of the excluded cases. Thus, dRSL must be significantly related to variability in both δ 18 O sanbao and MGSQ. In addition, the distributions of dRSL regression coefficients ( Supplementary Fig. 20 ) for both δ 18 O sanbao and MGSQ span intervals that do not cross zero, again implying that dRSL makes a significant contribution to the MLR models. Finally, it is important to note that synchronization of precession-band variance in RSL and δ 18 O sanbao ( Fig. 1e ) does not nullify the results of our MLR simulations with respect to the RSL component. The above synchronization is independent of both the amplitude of RSL variability and the timing of RSL variability at frequencies outside the precession bandwidth. Hence, it is only the potential effect of RSL variability on δ 18 O sanbao phasing in the precession band that cannot be examined in our simulation. We have already established, however, that the timing of δ 18 O sanbao variability in this bandwidth is closely coupled to that of Red Sea RSL (see previous sections and Supplementary Fig. 6b ). This relationship was determined using the ‘RSL dust-sanbao ’ chronology, which is unbiased by RSL-δ 18 O sanbao phase assumptions. Our new, radiometrically based and probabilistically assessed sea-level record enables—for the first time—reliable estimation of rates of sea-level change for the last 500 kyr that are unbiased by assumed phase relationships between changes in ice volume and other variables (for example, insolation, CO 2 , temperature), and unaffected by the (not insignificant) uncertainties associated with ice-core age modelling (unlike previous Red Sea RSL records [4] , [36] ). Our observations suggest that a global ice volume at least twice that of the present day (equivalent to ~−65 m sea level or lower) represents a critical threshold in ice-sheet development/decay. Our sea-level data therefore appear to corroborate and quantify previous hypotheses [37] and models [38] of increased ice-sheet instability at sufficiently large (‘excess’) ice volumes. Interestingly, increased ice-rafted detritus in deep-sea sediments at ~2.5 Myr (indicative of ice-sheet calving, hence, marine ice-sheet margins) has been linked to extension of the North American ice sheet to a point where it developed marine margins [39] , [40] . Global sea level stood at roughly −40 to −70 m at that time [41] , [42] , which is consistent with our inferred ~−65 m sea-level threshold. Possibly, therefore, the high potential rates of sea-level rise for ice volumes equivalent to 65 m sea-level fall ( Fig. 4a ) depend on the existence of marine margins. Regarding monsoon and ice-volume covariability, our results corroborate previous suggestions [6] , [10] , [17] , [43] that the extent of global glaciation strengthens/weakens the AWM/ASM. In addition, we find that dRSL is important for millennial-scale ASM and AWM variability, and for a lagged ASM response to insolation. For example, cross-spectral analyses of δ 18 O sanbao and our MLR models confirm previous suggestions that a lagged response of the ASM to insolation forcing (on orbital timescales) can be explained by the effects of northern hemisphere ice-volume changes on sensible heating of the Asian plateau [7] , [17] . At the millennial scale, glacial terminations have positive dRSL peaks and are associated with weak ASM and strong AWM events ( Fig. 3b,d,e ), and likely also with warm ‘overshoots’ in Antarctic temperature records [26] , [44] ( Fig. 3f ). This appears to portray a millennial-scale ‘bipolar see-saw’ event, where meltwater-related reduction of North Atlantic overturning circulation caused abrupt Northern Hemisphere cooling and widespread Southern Hemisphere warming [44] , [45] , with concomitant ASM weakening/failure [8] and AWM intensification [46] . In addition, our MLR simulations for MGSQ suggest that strong orbital cyclicity in late Pleistocene Chinese loess records [6] , [47] may reflect indirect orbital forcing via ice-sheet variability, rather than direct orbital control on the AWM. The RSL component carries an orbital signature, so we cannot infer the degree to which long-term AWM variability is a direct response to insolation forcing and/or the effects of ice-sheet changes on atmospheric circulation and land vegetation feedback processes. Palaeodata suggest that AWM intensity was strongly coupled to ice-volume changes over at least the past 1.1 Myr (ref. 48 ), while a modelling study suggests that AWM variability is a direct response to obliquity forcing through its effect on low–high latitude insolation gradients [49] . We note that the obliquity component is negligible in our results ( Supplementary Table 6 ). Differential latitudinal heating controls poleward heat and moisture fluxes, both of which are important in ice-sheet and Asian monsoon variability [50] , [51] . The relationship between AWM and ice-volume variability, and between their forcings and feedbacks, is therefore likely to be tightly coupled, hence deconvolving the components of orbital and ice-volume forcing from AWM records is not straightforward. Our results add to this endeavour by demonstrating that ice-volume changes alone can account for the combined orbital variance in a key AWM record. Our study, therefore, complements previous attempts to interpret Chinese cave speleothem δ 18 O in terms of Asian monsoon variability [8] , [17] , [52] , [53] , as well as AWM variability in terms of external (orbital) and internal (for example, ice volume) forcings [33] , [48] , [49] . Clearly, our simulations do not capture the total variance in δ 18 O sanbao or MGSQ, and in detail there are likely ice-volume ‘threshold effects’ on Asian monsoon dynamics [54] , hence other forcings and/or feedbacks may be important [17] , [34] , [48] . Nevertheless, the advantages of our approach are that it is grounded in real data, is chronologically unbiased by phase assumptions about benthic δ 18 O or ice-volume response to orbital parameters and that it quantitatively demonstrates that past fluctuations in global ice volume and its rates of change can account for much of the observed palaeomonsoon variability. Glacial isostatic modelling An extended version of the ICE-5G global ice model [31] was run over two complete glacial cycles, punctuated by a 4-kyr interglacial period with ice volume at near present-day values. The spherically symmetric, viscoelastic earth response is parameterized over three lithospheric thicknesses (71, 96 and 120 km), and over a discrete range of upper and lower mantle viscosities (1 × 10 20 to 1 × 10 21 Pa s and 2 × 10 21 to 5 × 10 22 Pa s, respectively). The glacial isostatic model was developed following principles outlined by Kendall et al . [55] Probabilistic assessment of Red Sea RSL record Chronological and vertical (sea-level) uncertainties for the RSL data (±12 m at 2 σ (refs 4 , 27 , 29 )) are combined for a Monte Carlo style, probabilistic assessment of RSL as described by Grant et al . [5] We also use this method to calculate the maximum probability (±2 σ ) of rates of sea-level change (dRSL) for the interval 150–500 kyr ( Fig. 4b ). Tests (not shown) using dRSL values derived straightforwardly from the raw RSL data reveal that peak ‘raw’ dRSL values are reasonably approximated by the upper bound of our 95% probability interval. For both the RSL and dRSL probabilistic assessments, we assume no covariance between sources of uncertainty. The probabilistic RSL and dRSL assessments for the interval 150–500 kyr are combined with similar probabilistic RSL and dRSL assessments for the last 150 kyr (ref. 5 ) which have more detailed age control ( Figs 2a and 3b ). Together, these give continuous, probabilistic records of sea-level variations and its rates of change over the last 500 kyr. MLR models Our MLR models for δ 18 O sanbao (Sanbao sim ) and Chinese loess (MGSQ sim ) use time series of the orbital components (eccentricity, E; precession, P; obliquity, O) [56] and our new, maximum-probability RSL and dRSL records. The MLR models can be expressed as: where bracketed values are bootstrap-derived s.e. We do not attach any quantitative meaning to the coefficients because we cannot rule out the possibility of multicollinearity in our regressions, and because time-series data-points are not independent. We therefore provide these factor loadings purely so that others can reproduce Sanbao sim and MGSQ sim . To investigate the validity of the dRSL component in these models, half of the data cases were selected at random. Using only the selected cases, a design matrix, X 0 , was constructed from E, O, P and RSL. An extended design matrix, X 1 , was then constructed based on the same cases with inclusion of dRSL. For the same cases in the given response variable (that is, δ 18 O sanbao or MGSQ), MLR coefficients were estimated using partial-least squares regressions (to reduce the influence of multicollinearity) on the basis of X 0 and X 1 . MLR fit quality was determined by the sum of squared errors (SSE) between the selected cases of the response variable and the corresponding MLR predicted responses. The fit improvement through the inclusion of dRSL in the model is expressed as the relative (%) reduction in SSE: Validation was then performed to test if inclusion of dRSL in the model produces a meaningful improvement (rather than one at random). On the basis of the estimated MLR coefficients, the cases excluded from X 0 and X 1 were used to predict the corresponding cases excluded from the response variable. Again, the quality of the predictions was assessed on the basis of SSE, and the relative improvement in the quality of the predictions was estimated in the same manner as the model improvement. The above process was repeated 10 4 times, with each iteration employing cases selected at random. The resulting distributions ( Supplementary Fig. 20 ) of regression coefficients, model improvements and prediction improvements provide a means to quantify the role of dRSL in the MLR model. The use of such a Monte Carlo approach obviates the need for traditional hypothesis testing, which can be compromised by the serial correlation typically exhibited in climate time series. How to cite this article : Grant, K. M. et al . Sea-level variability over five glacial cycles. Nat. Commun. 5:5076 doi: 10.1038/ncomms6076 (2014).